A narrow window of cortical tension guides asymmetric spindle positioning in the mouse oocyte Cell mechanics control the outcome of cell division. In mitosis, external forces applied on a stiff cortex direct spindle orientation and morphogenesis. During oocyte meiosis on the contrary, spindle positioning depends on cortex softening. How changes in cortical organization induce cortex softening has not yet been addressed. Furthermore, the range of tension that allows spindle migration remains unknown. Here, using artificial manipulation of mouse oocyte cortex as well as theoretical modelling, we show that cortical tension has to be tightly regulated to allow off-center spindle positioning: a too low or too high cortical tension both lead to unsuccessful spindle migration. We demonstrate that the decrease in cortical tension required for spindle positioning is fine-tuned by a branched F-actin network that triggers the delocalization of myosin-II from the cortex, which sheds new light on the interplay between actin network architecture and cortex tension. During mitosis, forces applied on the cortex by the cell environment can control spindle orientation [1] , [2] , but the cell itself generates forces essential for its division. Indeed, at mitosis onset, before centrosome separation, cells round up [3] following an increase in osmotic pressure [4] and an increase in cortical tension mediated by the cell cortex [3] , [5] . This process is essential to allow proper spindle morphogenesis, stability and positioning, as it creates an optimal volume for chromosome capture and allows interaction between the cell cortex and astral microtubules emanating from the centrosomes at spindle poles in all directions of the space [5] , [6] , [7] , [8] . In mouse oocytes on the contrary, off-center positioning of the spindle following its migration, required to allow the asymmetry in size of the first meiotic division, depends on a reduced cortical tension which is correlated with both increased cortical actin nucleation and myosin-II delocalization from the cell cortex [9] . Mouse oocytes are arrested in Prophase I of the first meiotic division (Meiosis I) in the ovary. Upon hormonal stimulation meiosis resumes, triggering Nuclear Envelope BreakDown (NEBD) and the two consecutive meiotic divisions. Rapidly, the first meiotic spindle forms, rarely at the perfect cell center but slightly off-centered [10] , [11] . At that stage, the oocyte bears no apparent sign of polarization [12] , [13] , [14] . The spindle then migrates along its long axis towards the closest cortex [10] . Mouse oocytes lacking true centrosomes and astral microtubules [15] , spindle positioning in female mouse meiosis does not depend on microtubules [10] as in mitosis where astral microtubules connect the spindle to the cortex to actively position it within the cell [8] . Spindle positioning in Meiosis I instead depends on the progressive assembly of two actin networks: a cytoplasmic meshwork nucleated by Formin-2 (refs 16 , 17 , 18 , 19 ) and Spire1/2 (ref. 20 ) together with a cortical actin thickening nucleated by the Arp2/3 complex [9] . Mos, a MAPKKK (MAP Kinase Kinase Kinase) expressed specifically in oocytes after NEBD and activating MAPKs around 3 h after NEBD [10] , [21] , [22] controls both the nucleation of this actin thickening and the removal of myosin-II from the cortex, two events responsible for the drop in cortical tension required for spindle migration [9] , [23] . However, to which extent and why cortical tension needs to decrease in mouse oocytes to trigger spindle migration has so far remained elusive. Here using mathematical modelling and cortical tension manipulation, we show that cortical tension is strictly gated to allow spindle migration and that the decrease in cortical tension is mediated by F-actin dependent myosin-II exclusion from the cortex. Spindle position correlates with F-actin density asymmetry To investigate how the regulation of cortical tension affects spindle movement to the cortex, we developed a theoretical model of spindle migration based on the following observations. During spindle positioning, F-actin forms an actin cage that surrounds the microtubule spindle and connects it to the thick actin cortex [18] , [19] ( Fig. 1a ). At that stage, myosin-II is located at both spindle poles [19] , [24] and its inhibition impairs spindle migration [9] , [19] . In addition, a local stretching of the cortical actin thickening can be observed at the cortex above the approaching spindle pole [9] ( Figs 1a , 2a ). This suggests that myosin-II pulls the spindle towards the cortex from both poles by pulling on filaments emanating from the cortical thickening overlapping with filaments emanating from the actin cage. Therefore, the pulling force should depend on the overlap between cortical and cytoplasmic filaments, which should be more important on the side where the spindle is migrating, accounting for the directionality of spindle migration [10] , [11] . 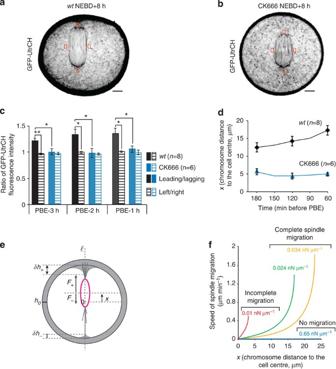Figure 1: The actin cage is pulled towards the cortex during Meiosis I. (a,b) Confocal spinning disk images of awtoocyte untreated (a) and treated with 200 μM of CK666 (b). Oocytes are in late Meiosis I (NEBD+8 h), they express GFP-UtrCH (black), one Z-plane is shown and the orange rectangles highlight the regions taken to measure the density of actin filaments depicted inc. Scale bars: 10 μm. (c) Ratio of GFP-UtrCH fluorescence intensity between regions taken above the leading and lagging spindle poles (full bars), and between the left and right side of the spindle (striped bars). Measurements were taken in eightwtoocytes (black bar) and sixwtoocytes treated with CK666 (blue bar) 3, 2 and 1 h before polar body extrusion (PBE). Mean is shown over three independent experiments. Standard error of the mean is plotted on each bar. Statistical difference is assessed with at-test or at-test with Welch correction (P-values: PBE-3 h,wtleading/lagging versus left/right 0.0032,wtversus CK666 0.0215; PBE-2 h:wtleading/lagging versus left/right 0.0132,wtversus CK666 0.0275; PBE-1 h:wtleading/lagging versus left/right 0.0156,wtversus CK666 0.0469). There is no difference between left/right fluorescence intensities at all stages in all conditions and between leading/lagging fluorescence intensities of oocytes treated with CK666 (Kruskal–Wallis test,P-value=0.1024). (d) Graph showingx, the chromosome distance to the cell center, as a function of time before PBE, for eightwtoocytes (black) and sixwtoocytes treated with CK666 (blue). Mean is shown over three independent experiments. Standard error of the mean is plotted on each point. (e) Model of spindle migration. The pink object represents the spindle andxthe position of the chromosomes at a given timet. Actin is in grey. The spindle poles are source of actin polymerization (dark grey lines).h0represents the cortical actin thickening,δh+the local stretching of the cortical actin thickening above the leading pole andδh−on the other side.F+andF−are the pulling forces exerted on the spindle poles. (f) Model prediction of spindle velocityas a function of chromosome position for increasing values of cortical tensionk. Figure 1: The actin cage is pulled towards the cortex during Meiosis I. ( a , b ) Confocal spinning disk images of a wt oocyte untreated ( a ) and treated with 200 μM of CK666 ( b ). Oocytes are in late Meiosis I (NEBD+8 h), they express GFP-UtrCH (black), one Z-plane is shown and the orange rectangles highlight the regions taken to measure the density of actin filaments depicted in c . Scale bars: 10 μm. ( c ) Ratio of GFP-UtrCH fluorescence intensity between regions taken above the leading and lagging spindle poles (full bars), and between the left and right side of the spindle (striped bars). Measurements were taken in eight wt oocytes (black bar) and six wt oocytes treated with CK666 (blue bar) 3, 2 and 1 h before polar body extrusion (PBE). Mean is shown over three independent experiments. Standard error of the mean is plotted on each bar. Statistical difference is assessed with a t -test or a t -test with Welch correction ( P -values: PBE-3 h, wt leading/lagging versus left/right 0.0032, wt versus CK666 0.0215; PBE-2 h: wt leading/lagging versus left/right 0.0132, wt versus CK666 0.0275; PBE-1 h: wt leading/lagging versus left/right 0.0156, wt versus CK666 0.0469). There is no difference between left/right fluorescence intensities at all stages in all conditions and between leading/lagging fluorescence intensities of oocytes treated with CK666 (Kruskal–Wallis test, P -value=0.1024). ( d ) Graph showing x , the chromosome distance to the cell center, as a function of time before PBE, for eight wt oocytes (black) and six wt oocytes treated with CK666 (blue). Mean is shown over three independent experiments. Standard error of the mean is plotted on each point. ( e ) Model of spindle migration. The pink object represents the spindle and x the position of the chromosomes at a given time t . Actin is in grey. The spindle poles are source of actin polymerization (dark grey lines). h 0 represents the cortical actin thickening, δh + the local stretching of the cortical actin thickening above the leading pole and δh − on the other side. F + and F − are the pulling forces exerted on the spindle poles. ( f ) Model prediction of spindle velocity as a function of chromosome position for increasing values of cortical tension k . 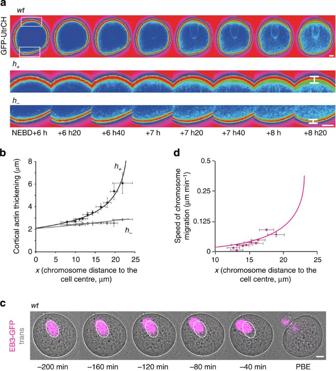Figure 2: The force exerted on the spindle is converted into a movement towards the cortex. (a) Upper panel: confocal spinning disk images of awtoocyte in late Meiosis I expressing GFP-UtrCH (blue, lowest intensity; red, highest intensity). One Z-plane is shown. Scale bar: 10 μm. Frames are 20 min apart. Lower panel: magnifications of the white boxes presented in the upper panel. The white bars indicateh+(top) andh−(bottom). Scale bar: 3 μm. (b) Quantification of the deformation of the cortex (h+: black dots,h−: grey dots) in μm as a function of chromosome positionxin μm and corresponding fitted curves (black and grey). Quantification starts at NEBD+6 h. Mean of 10 oocytes over three different experiments is shown. Standard error of the mean is shown. (c) Confocal spinning disk images of awtoocyte in late Meiosis I expressing EB3-GFP (pink). A Z-projection over 20 μm is shown. Time is given in minutes before polar body extrusion (PBE). The white ellipsoid highlights the initial position of the spindle. Scale bar: 10 μm. (d) Speed of the spindle as a function of chromosome positionx(pink dots) and corresponding fitted curve (pink). Mean of 12 oocytes is shown from four independent experiments. Standard error of the mean is plotted. Full size image Figure 2: The force exerted on the spindle is converted into a movement towards the cortex. ( a ) Upper panel: confocal spinning disk images of a wt oocyte in late Meiosis I expressing GFP-UtrCH (blue, lowest intensity; red, highest intensity). One Z-plane is shown. Scale bar: 10 μm. Frames are 20 min apart. Lower panel: magnifications of the white boxes presented in the upper panel. The white bars indicate h + (top) and h − (bottom). Scale bar: 3 μm. ( b ) Quantification of the deformation of the cortex ( h + : black dots, h − : grey dots) in μm as a function of chromosome position x in μm and corresponding fitted curves (black and grey). Quantification starts at NEBD+6 h. Mean of 10 oocytes over three different experiments is shown. Standard error of the mean is shown. ( c ) Confocal spinning disk images of a wt oocyte in late Meiosis I expressing EB3-GFP (pink). A Z-projection over 20 μm is shown. Time is given in minutes before polar body extrusion (PBE). The white ellipsoid highlights the initial position of the spindle. Scale bar: 10 μm. ( d ) Speed of the spindle as a function of chromosome position x (pink dots) and corresponding fitted curve (pink). Mean of 12 oocytes is shown from four independent experiments. Standard error of the mean is plotted. Full size image To test this hypothesis, we measured the fluorescence intensity of the F-actin probe (GFP-UtrCH) [25] as a proxy for filament density throughout spindle migration. We measured it between the nearest spindle pole from the cortex (leading pole) and the cortex above it, between the opposite spindle pole (lagging pole) and the cortex below it and on the sides of the spindle ( Fig. 1a orange rectangles). We found that the fluorescence intensity of GFP-UtrCH is higher between the leading pole and its above cortex than between the lagging pole and its nearest cortex ( Fig. 1c , the ‘leading/lagging’ ratios represented as black bars are always above 1). This difference can be observed throughout spindle migration ( Fig. 1c,d back dots). It suggests that during spindle migration the overlap between cortical and cytoplasmic filaments is indeed larger between the leading pole and its above cortex than between the lagging pole and its nearest cortex. It is fully consistent with FRAP measurements of actin-YFP performed in these two regions at that stage that also show an increase in more stable F-actin above the leading spindle pole [18] . In addition, when the spindle stays centrally located ( Fig. 1b,d blue triangles) after inhibition of the Arp2/3 complex in oocytes using CK666 (refs 9 , 26 ), leading to an absence of cortical actin thickening [9] , the asymmetry in actin density between the leading and lagging poles is completely abolished as the ratios during the same period of time are always close to 1 ( Fig. 1c blue bars). Thus, when the spindle remains centrally located, there is no asymmetry in the distribution of actin filaments ( Fig. 1c ). This strongly argues for a dependency between spindle position and the size of overlap between cortical and cytoplasmic filaments, and thus pulling strength. Consistent with this, as the spindle migrates and the overlap at the leading pole increases, the pulling force should build up resulting in the acceleration of spindle speed. This is precisely what we observe, as the speed of spindle migration increases when it approaches the cortex [10] ( Fig. 2d ). In all conditions and at all time points, the actin density is similar on both sides of the spindle ( Fig. 1c striped bars). Furthermore, for control oocytes, the actin density is similar on spindle sides and close to the lagging pole of the spindle ( Supplementary Fig. 1a ), arguing against a pushing mechanism from the rear of the spindle [27] at least at that stage. Model prediction on cortical tension To account for these observations, we modelled the spindle in one dimension as an ellipsoid whose center of mass is moving along its long axis under pulling forces exerted at each pole ( F + at the leading pole and F − at the lagging pole) ( Fig. 1e ). Actin filaments emanate from the actin cage at spindle poles and from the overlying cortex, creating the overlap [9] ( Figs 1a , 2a ). The density of actin filaments is plotted in Supplementary Fig. 1b . Cytoplasmic filaments can penetrate the cortex and vice-versa, cortical filaments can be extracted from the cortex (creating a local deformation of the cortical actin thickening). Both events depend on cortical tension and/or actin density that is also related to cortex tension. Assuming that the cytoplasmic filaments grow slower when they penetrate the cortex, in accordance with the fact that cortical and cytoplasmic actin define two different compartments in terms of dynamics [9] , we can postulate that the mean length of filaments in the cortex depends on how fast they can grow against the load of cortical tension. Thus, it should be directly affected by cortical tension (see Methods section). Conversely, cortical filaments should be more easily extracted from the cortex if the tension is low than if it is high, which leads to a similar dependence of cortex deformability on cortical tension. Solving analytically the model for different values of cortical tension leads to a phase diagram showing that cortical tension has a narrow permissive window into which it must fall to allow spindle migration ( Fig. 1f ). The model thus predicts that if cortical tension is too high, the spindle would not migrate ( Fig. 1f blue curve). One explanation could be that cytoplasmic filaments emanating from the actin cage would have more difficulty to penetrate into the cortex and cortical filaments would be less extracted from the cortex, reducing the region of overlap. This is indeed what we observe ( Fig. 1b–d , CK666-treated oocytes, Supplementary Fig. 2 ) and what was previously shown [9] ( Fig. 1f blue curve, 0.65 nN μm −1 corresponds to the value of cortical tension measured by micropipette aspiration in mos−/− oocytes, lacking cortical thickening and impaired for off-center spindle positioning [9] ). Unexpectedly, the model additionally predicts that if the cortex is too soft, spindle migration would also be impaired ( Fig. 1f red curve). Indeed if too soft, the cortex would not support the pulling force and would break up as the spindle approaches. Therefore, the main prediction from the model is that cortical tension has to be tightly gated in oocytes to allow spindle migration ( Fig. 1f yellow curve, 0.034 nN μm −1 corresponds to the value of cortical tension measured in control oocytes where migration does occur [9] ). Before testing this prediction, we verified that the model actually reflects our experimental measurements. The model is consistent with experimental measurements We first calculated an estimate of the forces exerted on each poles of the spindle ( F + and F − ) in late Meiosis I when the spindle has almost finished its migration (using x =17 μm, x representing the chromosome distance to the cell center). These forces, responsible for spindle displacement to the cortex and local stretching of the cortical actin thickening ( Figs 1a , 2a ), depend on the elastic response of the cortex through the spring constant k sp and on the cortical actin-thickening deformation δh ( Fig. 1e δh + above the leading pole and δh − above the lagging pole) such that F ± = k sp δh ± . The total force F tot is then the difference between these two forces ( F tot = F + – F − ). k sp can be estimated by the cortical tension k , measured at 0.034 nN μm −1 in wt oocytes during late Meiosis I [9] . We then measured the cortical actin-thickening deformation δh above each pole of the spindle ( δh + is visible in 92.3% of the cases, whereas δh − is never detectable). Above the leading pole, the cortical actin thickening h + = h o + δh + ( Fig. 1e ) increases from 3 to 6 μm between NEBD+6 h and NEBD+8 h ( Fig. 2a,b black dots). In late Meiosis I when x =17 μm, we measured h + =4.5 μm and h o =3 μm ( Fig. 2b black dots), leading to δh + ≈1.5 μm. Using F + = k sp δh + , we calculate an estimate of F + ≈0.05 nN. Above the lagging pole, the cortical actin thickening h − = h o + δh − remains roughly constant after NEBD+6 h until NEBD+8 h ( Fig. 2b grey dots). In late Meiosis I when x =17 μm, h − ≈ h o ( Fig. 2b ), leading to δh − ≈0 μm, within measurement error. Thus F − is close to 0 nN and negligible compared with F + . Hence the total force ( F tot = F + – F − ) exerted on the spindle in late Meiosis I is ~0.05 nN. This is a weak force (a single myosin molecule exerts a force in the range of 3–4 pN [28] ), but the spindle moves very slowly towards the cortex inside the cell at a mean speed of 0.15 μm min −1 in late Meiosis I [19] . In comparison, in oocytes treated with CK666 ( Fig. 1b ), cortical thickness remains constant at 1.5 μm ( Supplementary Fig. 2a ), leading to F + = F − and to an absence of spindle migration ( Supplementary Fig. 2b ). Using the equation for the actin distribution that we established (see Methods section), we solved it analytically for δh + and δh − ( Fig. 2b black and grey curves) using these known values: h 0 =3 μm (as measured in Fig. 2a,b black and grey dots), L =17 μm ( L is the distance between the leading pole and its above cortex when it starts migrating as measured in refs 10 and 19 ) and k =0.034 nN μm −1 (cortical tension measured by micropipette aspiration in ref. 9 ). It yields values for ℓ 0 of 7 μm ( ℓ 0 is the mean length of actin filaments in the cytoplasm), very close from what was measured in ref. 19 , and for ℓ c of 0.5 μm ( ℓ c is the mean length of actin filaments penetrating the cortex) in the proper range for cortical filaments, h o measuring ~3 μm ( Fig. 2a,b black and grey dots). Furthermore, using this fit, we can extract an order of magnitude of the stall cortical tension ( k stall ), that is, the tension at which the cortex does not allow the growth of cytoplasmic actin filaments. From the fitting, k stall is in the range of 0.01 nN μm −1 , close to 0.034 nN μm −1 , the value of cortical tension measured by micropipette aspiration in control oocytes [9] . This means that above a cortical tension roughly in this range, the cytoplasmic actin filaments cannot enter the cortex. Hence, when the tension is too high, the overlap between cortical and cytoplasmic filaments is impaired and the spindle will not migrate, which is the case when the tension is one order of magnitude higher (case of mos−/− oocytes lacking a cortical thickening and impaired for off-center spindle positioning [9] ). Another way to calculate an estimate of the forces exerted at spindle poles is to use the force balance to describe the total force F tot as a function of the spindle speed tempered by the viscous drag γ exerted by the cytoplasm of the cell: . The speed of spindle migration was measured and plotted as a function of chromosome position x ( Fig. 2c,d pink dots). Imputing the same known values as for Fig. 2b ( h 0 =3 μm as measured in Fig. 2b , L =17 μm as measured in refs 10 and 19 [19] , k =0.034 nN μm −1 as measured in ref. 9 ), we fitted the speed as a function of time ( Fig. 2d pink curve). We obtain a friction parameter γ =2 nN min μm −1 , which, for a spindle of roughly 30 μm in length [29] and 15 μm in width [30] gives a total viscosity of 6 × 10 2 Pa s. To further test the match between our model and our observations, we measured the viscosity η in late Meiosis I oocytes using micropipette aspiration (see Methods section, Supplementary Fig. 1c,d ). We obtain a value of viscosity of 1.6 × 10 2 ±0.5 Pa s in the same range as other cell types measured using the same technique [31] and close to the calculated value of 6 × 10 2 Pa s. Altogether our model yields calculated values of force, filament length and viscosity in the same range as our experimental measurements or known values from the literature. Thus, we decided to test its prediction. The cortical F-actin thickening chases cortical myosin-II The main prediction of the model is that the window of cortical tension allowing spindle migration is narrow ( Fig. 1f ). We have shown previously that a high cortical tension impairs spindle migration [9] , we thus investigated whether a low cortical tension would have the same effect ( Fig. 1f red curve). To test this, we tried to further decrease cortical tension during Meiosis I. The drop in cortical tension required for Meiosis I spindle migration correlates with myosin-II displacement from the cortex and with the nucleation of a cortical actin thickening by the Arp2/3 complex [9] . We therefore fused the VCA domain of Wave2, a nucleating promoting factor that activates Arp2/3 (ref. 32 ), to ezrin (Ez), a member of the ERM (ezrin-radixin-moesin) family located at the cortex of mouse oocytes [33] (whole construct referred below as cVCA for cortical VCA). This allowed us to target the VCA domain and activate the Arp2/3 complex [34] , specifically at the oocyte cortex. The cVCA is mostly enriched at the cortex throughout Meiosis I ( Supplementary Fig. 3a,d ). We then visualized cortical actin in Prophase I at a stage where MAPKs are not activated, as their activator, Mos, is not yet expressed [35] , [21] . Targeting the VCA to the plasma membrane is sufficient to nucleate de novo an actin thickening independently of the Mos/MAPK pathway ( Fig. 3a compare upper and lower panels). To assess cortical actin thickness in Prophase I oocytes expressing the cVCA, we measured the overall thickness of the outer bright layer (the only one present in Prophase I control oocytes) and the inner dimmer layer ( Fig. 3a orange dashes). In control Prophase I oocytes, cortical actin thickness is stable over time staying around 1.7 μm wide ( Fig. 3b,c black curve), whereas in oocytes expressing the cVCA, it reaches progressively to a maximum of 3.5 μm ( Fig. 3b,c red curve). Furthermore and very surprisingly, it is also sufficient to chase myosin-II from the cortex ( Fig. 3d compare upper and lower panels). Indeed, we followed endogenous myosin-II localization using a specific GFP-coupled intrabody directed against myosin-II [36] and measured the ratio between the average fluorescence signal intensity in the cortex versus the cytoplasm. If the ratio is above 1, then myosin-II is cortically enriched, whereas if it is below 1, it is enriched in the cytoplasm. Myosin-II is clearly cortically enriched in control oocytes ( Fig. 3e black bar) [9] , whereas it is not in oocytes expressing the cVCA ( Fig. 3e red bar). Taken together, these results show that the nucleation of cortical actin filaments by the Arp2/3 complex is sufficient to trigger by itself the delocalization of myosin-II from the cortex, independently of the Mos/MAPK pathway. None of these effects are due to the presence of Ez in the construct, as oocytes simply overexpressing Ez ( Supplementary Fig. 3g ) do not trigger an ectopic actin thickening ( Fig. 3c grey curve) or myosin-II removal from the cortex ( Fig. 3e grey bar). Importantly, the expression of the cVCA in Prophase I oocytes impairs neither the overall architecture of the cytoplasmic actin meshwork present at that stage [20] , [37] , [38] ( Supplementary Fig. 3e ) nor its dynamics, as the vesicles present at the crossing points of actin filaments move at a speed of 12.4±3.8 μm min −1 ( Supplementary Movie 1 ), similarly to the speed of 12.8±3.4 μm min −1 previously reported [38] . Cell cycle progression is not deeply affected by expression of the cVCA or Ez, as anaphase occurs in both cases at around the same time as in controls ( Supplementary Fig. 4a ). Interestingly, most cVCA-expressing oocytes attempt to extrude a polar body on time ( Supplementary Fig. 4b ), but often with a bleb-like configuration or subsequent retraction of their polar body, suggesting that the important deformation of the oocyte following cVCA expression ( Fig. 3g lower panel) provokes a spatial proximity between the oocyte cortex and the chromosomes, which is sufficient to induce polar body extrusion. 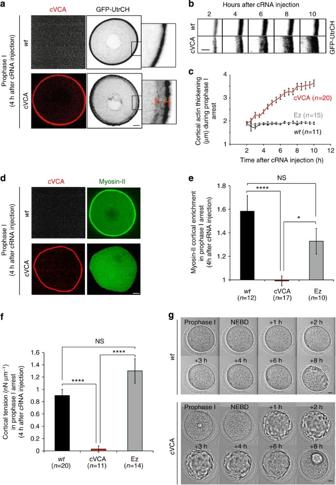Figure 3: The cortical actin thickening is responsible for myosin-II exclusion from the cortex and decrease in cortical tension in Meiosis I. (a) Confocal spinning disk images of Prophase I oocytes expressing GFP-UtrCH (black) alone (upper panel) or together with cVCA (red) (bottom panel), observed 4 h after cRNA injection. Boxes represent magnification of the cortical region. Orange dashes represent cortical actin thickness measured inc. One Z-plane is shown. Scale bar: 10 μm. (b) Time-lapse spinning disk confocal images of the cortex of awtoocyte expressing GFP-UtrCH (black) alone (upper panel) or together with cVCA (red) (bottom panel) during Prophase I, observed from 2 h after cRNA injection until 10 h. One Z-plane is shown. Scale bar: 4 μm. (c) Curves showing cortical actin thickness as a function of time after cRNA injection during Prophase I. Mean is shown of 11 oocytes expressing GFP-UtrCH alone (black curve), 20 oocytes expressing also cVCA (red curve) and 15 oocytes expressing also Ez (grey curve) assessed over two independent experiments. Standard error of the mean is shown. (d) Confocal spinning disk images of a Prophase I oocyte expressing SF9-GFP (myosin-II intrabody, green) alone (upper panel) or together with cVCA (red) (bottom panel), observed 4 h after cRNA injection. One Z-plane is shown. Scale bar: 10 μm. (e) Bar graph showing the ratio between the average intensities of cortical versus cytoplasmic myosin-II in Prophase I oocytes after 4 h of expression of SF9-GFP alone (black bar,n=12 oocytes), SF9-GFP and cVCA (red bar,n=17 oocytes), or SF9-GFP and Ez (grey bar,n=15 oocytes). For each oocyte, six measurements were taken in the cortex and six in the cytoplasm. Mean is shown assessed over three independent experiments. Standard error is plotted on each bar. The statistical significance of differences is assessed with at-test or at-test with Welch correction (P-values: SF9-GFP-expressing oocytes versus SF9-GFP and cVCA-expressing oocytes 0.0002; SF9-GFP-expressing oocytes versus SF9-GFP and Ez-expressing oocytes 0.609; SF9-GFP and Ez-expressing oocytes versus SF9-GFP and cVCA-expressing oocytes 0.0145). (f) Bar graph showing values of cortical tension in Prophase I oocytes (black bar, minimum value see Method section,n=20 oocytes), Prophase I oocytes expressing cVCA (red bar,n=11 oocytes) or Ez (grey bar, minimum value see Method section,n=14 oocytes) measured 4 h after cRNA injection. Mean is shown, assessed over two independent experiments. Standard error is plotted on each bar. Statistical differences were assessed with at-test with Welch correction (P-values:wtoocytes versus cVCA-expressing oocytes <0.0001;wtoocytes versus Ez-expressing oocytes 0.0892; Ez-expressing oocytes versus cVCA-expressing oocytes <0.0001). (g) Confocal spinning disk transmitted light images of awtoocyte or awtoocyte expressing cVCA during Meiosis I. At the time point Prophase I, oocytes have expressed cRNAs for 2 h, they undergo NEBD 1 h later. Scale bar: 10 μm. Figure 3: The cortical actin thickening is responsible for myosin-II exclusion from the cortex and decrease in cortical tension in Meiosis I. ( a ) Confocal spinning disk images of Prophase I oocytes expressing GFP-UtrCH (black) alone (upper panel) or together with cVCA (red) (bottom panel), observed 4 h after cRNA injection. Boxes represent magnification of the cortical region. Orange dashes represent cortical actin thickness measured in c . One Z-plane is shown. Scale bar: 10 μm. ( b ) Time-lapse spinning disk confocal images of the cortex of a wt oocyte expressing GFP-UtrCH (black) alone (upper panel) or together with cVCA (red) (bottom panel) during Prophase I, observed from 2 h after cRNA injection until 10 h. One Z-plane is shown. Scale bar: 4 μm. ( c ) Curves showing cortical actin thickness as a function of time after cRNA injection during Prophase I. Mean is shown of 11 oocytes expressing GFP-UtrCH alone (black curve), 20 oocytes expressing also cVCA (red curve) and 15 oocytes expressing also Ez (grey curve) assessed over two independent experiments. Standard error of the mean is shown. ( d ) Confocal spinning disk images of a Prophase I oocyte expressing SF9-GFP (myosin-II intrabody, green) alone (upper panel) or together with cVCA (red) (bottom panel), observed 4 h after cRNA injection. One Z-plane is shown. Scale bar: 10 μm. ( e ) Bar graph showing the ratio between the average intensities of cortical versus cytoplasmic myosin-II in Prophase I oocytes after 4 h of expression of SF9-GFP alone (black bar, n =12 oocytes), SF9-GFP and cVCA (red bar, n =17 oocytes), or SF9-GFP and Ez (grey bar, n =15 oocytes). For each oocyte, six measurements were taken in the cortex and six in the cytoplasm. Mean is shown assessed over three independent experiments. Standard error is plotted on each bar. The statistical significance of differences is assessed with a t -test or a t -test with Welch correction ( P -values: SF9-GFP-expressing oocytes versus SF9-GFP and cVCA-expressing oocytes 0.0002; SF9-GFP-expressing oocytes versus SF9-GFP and Ez-expressing oocytes 0.609; SF9-GFP and Ez-expressing oocytes versus SF9-GFP and cVCA-expressing oocytes 0.0145). ( f ) Bar graph showing values of cortical tension in Prophase I oocytes (black bar, minimum value see Method section, n =20 oocytes), Prophase I oocytes expressing cVCA (red bar, n =11 oocytes) or Ez (grey bar, minimum value see Method section, n =14 oocytes) measured 4 h after cRNA injection. Mean is shown, assessed over two independent experiments. Standard error is plotted on each bar. Statistical differences were assessed with a t -test with Welch correction ( P -values: wt oocytes versus cVCA-expressing oocytes <0.0001; wt oocytes versus Ez-expressing oocytes 0.0892; Ez-expressing oocytes versus cVCA-expressing oocytes <0.0001). ( g ) Confocal spinning disk transmitted light images of a wt oocyte or a wt oocyte expressing cVCA during Meiosis I. At the time point Prophase I, oocytes have expressed cRNAs for 2 h, they undergo NEBD 1 h later. Scale bar: 10 μm. Full size image Overdecreasing cortical tension impairs spindle migration cVCA expression induces a major decrease in cortical tension, measured using the micropipette aspiration technique at 0.03 nN μm −1 in Prophase I cVCA-expressing oocytes ( Fig. 3f red bar) versus 0.9 nN μm −1 minimum (see Methods section) in controls ( Fig. 3f black bar). As a consequence, these oocytes are deformed and no longer round nor stable in shape like controls ( Fig. 3g compare upper and lower panels, Supplementary Movies 2,3 , Supplementary Fig. 3c ), arguing that cortical tension further decreases as Meiosis I proceeds. This is not due to the presence of Ez in the fusion construct, a oocytes overexpressing only Ez harbour a minimal tension of 1.3 nN μm −1 in Prophase I, comparable to the tension measured in controls ( Fig. 3f grey bar). To test whether a very low cortical tension impacts spindle migration ( Fig. 1f red curve), we expressed the cVCA in wt oocytes, let them progress into Meiosis I and followed their chromosomes. cVCA expression prevents spindle migration in 92% of the cases compared with a basal level of 15% in controls ( Fig. 4a,b , Supplementary Movies 2,3 ). This again is not due to the presence of Ez, as oocytes overexpressing it harbour an incomplete or lack of spindle migration in only 29% of the cases, not statistically different from the controls ( Fig. 4b ), even though the cortical enrichment of Ez is higher than the one of the cVCA ( Supplementary Fig. 3g ). The dismantlement of the cytoplasmic actin meshwork, which normally occurs at NEBD [37] , does take place in oocytes expressing the cVCA ( Fig. 4c,d , Supplementary Movie 1 . Note that the ectopic cortical thickening is not yet detectable in Fig. 4c , as oocytes are observed 2 h after cRNA injection, as shown in Fig. 3c ). This excludes any stabilization effect of cytoplasmic F-actin at NEBD to account for the absence of spindle migration. The lack of spindle migration is then clearly due to a very low cortical tension throughout Meiosis I, which is consistent with the prediction from the model. 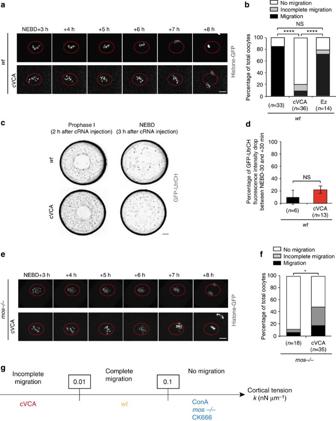Figure 4: Cortical tension has to be tightly regulated to allow spindle migration. (a) Confocal spinning disk images ofwtoocytes in Meiosis I expressing Histone-GFP (white) alone (upper panel) or together with cVCA (lower panel). Frames are 1 h apart. At NEBD, oocytes have expressed cRNAs for 3 h. A Z-projection over 20 μm is shown. The red circle highlights the initial position of the chromosomes before migration. Scale bar: 10 μm. (b) Bar graph representing the percentage of oocytes out of 33 Prophase I oocytes, 36 Prophase I oocytes expressing cVCA or 14 expressing Ez undergoing normal spindle migration (black bar), incomplete spindle migration (grey bar) or no spindle migration (white bar) over four independent experiments. At NEBD, oocytes have expressed cRNAs for 3 h. Statistical difference of repartition was assessed using aχ2-test (P-values:wtoocytes versus cVCA-expressing oocytes <0.0001;wt oocytes versus Ez-expressing oocytes 0.2849; Ez-expressing oocytes versus cVCA-expressing oocytes <0.0001). (c) Confocal spinning disk images of awtoocyte expressing GFP-UtrCH (black) alone (upper panel) or together with cVCA (lower panel) 2 h (Prophase I) and 3 h (NEBD) after cRNA injection, when the actin thickening is not yet formed (seeFig. 3c). Scale bar: 10 μm. (d) Bar graph representing the percentage of GFP-UtrCH fluorescence intensity drop between NEBD-30 min (2 h 30 min after cRNA injection) and NEBD+30 min (3h 30 min after cRNA injection) in 6wtoocytes (black bar) and 13wtoocytes expressing cVCA (red bar) over three independent experiments. Mean is shown. Standard error of the mean is plotted. Statistical difference was assessed using at-test (P-value=0.0995). (e) Confocal spinning disk images ofmos−/−oocytes in Meiosis I expressing Histone-GFP (white) alone (upper panel) or together with cVCA (lower panel). At NEBD, oocytes have expressed cRNAs for 3 h. Frames are 1 h apart. A Z-projection over 20 μm is shown. The red circle highlights the initial position of the chromosomes before migration. Scale bar: 10 μm. (f) Bar graph representing the percentage of oocytes out of 11mos−/−oocytes or 23mos−/−oocytes expressing cVCA undergoing normal (black bar), incomplete (grey bar) or no spindle migration (white bar) over five independent experiments. At NEBD, oocytes have expressed cRNAs for 3 h. Statistical difference of repartition was assessed using aχ2-test (P-value=0.0235). If we group the oocytes harboring either an incomplete or complete spindle migration in both conditions, theP-value=0.0077 using a Fisher test. (g) Schematic representing spindle migration as a function of measured cortical tension in mouse oocytes. ConA: oocytes treated with 100 μg ml−1of Concanavalin A, see ref.9. CK666: oocytes treated with 200 μM of CK666, see ref.9. Figure 4: Cortical tension has to be tightly regulated to allow spindle migration. ( a ) Confocal spinning disk images of wt oocytes in Meiosis I expressing Histone-GFP (white) alone (upper panel) or together with cVCA (lower panel). Frames are 1 h apart. At NEBD, oocytes have expressed cRNAs for 3 h. A Z-projection over 20 μm is shown. The red circle highlights the initial position of the chromosomes before migration. Scale bar: 10 μm. ( b ) Bar graph representing the percentage of oocytes out of 33 Prophase I oocytes, 36 Prophase I oocytes expressing cVCA or 14 expressing Ez undergoing normal spindle migration (black bar), incomplete spindle migration (grey bar) or no spindle migration (white bar) over four independent experiments. At NEBD, oocytes have expressed cRNAs for 3 h. Statistical difference of repartition was assessed using a χ 2 -test ( P -values: wt oocytes versus cVCA-expressing oocytes <0.0001; w t oocytes versus Ez-expressing oocytes 0.2849; Ez-expressing oocytes versus cVCA-expressing oocytes <0.0001). ( c ) Confocal spinning disk images of a wt oocyte expressing GFP-UtrCH (black) alone (upper panel) or together with cVCA (lower panel) 2 h (Prophase I) and 3 h (NEBD) after cRNA injection, when the actin thickening is not yet formed (see Fig. 3c ). Scale bar: 10 μm. ( d ) Bar graph representing the percentage of GFP-UtrCH fluorescence intensity drop between NEBD-30 min (2 h 30 min after cRNA injection) and NEBD+30 min (3h 30 min after cRNA injection) in 6 wt oocytes (black bar) and 13 wt oocytes expressing cVCA (red bar) over three independent experiments. Mean is shown. Standard error of the mean is plotted. Statistical difference was assessed using a t -test ( P -value=0.0995). ( e ) Confocal spinning disk images of mos−/− oocytes in Meiosis I expressing Histone-GFP (white) alone (upper panel) or together with cVCA (lower panel). At NEBD, oocytes have expressed cRNAs for 3 h. Frames are 1 h apart. A Z-projection over 20 μm is shown. The red circle highlights the initial position of the chromosomes before migration. Scale bar: 10 μm. ( f ) Bar graph representing the percentage of oocytes out of 11 mos−/− oocytes or 23 mos−/− oocytes expressing cVCA undergoing normal (black bar), incomplete (grey bar) or no spindle migration (white bar) over five independent experiments. At NEBD, oocytes have expressed cRNAs for 3 h. Statistical difference of repartition was assessed using a χ 2 -test ( P -value=0.0235). If we group the oocytes harboring either an incomplete or complete spindle migration in both conditions, the P -value=0.0077 using a Fisher test. ( g ) Schematic representing spindle migration as a function of measured cortical tension in mouse oocytes. ConA: oocytes treated with 100 μg ml −1 of Concanavalin A, see ref. 9 . CK666: oocytes treated with 200 μM of CK666, see ref. 9 . Full size image Our model also predicts that a high cortical tension prevents spindle migration ( Fig. 1f blue curve). This is indeed the case [9] , as in mos−/− oocytes, where cortical tension stays high throughout Meiosis I [9] , spindle migration is impaired [10] . We decided to test whether we could rescue spindle migration in these oocytes by simply decreasing their cortical tension after expression of the cVCA. Because this construct is very potent in decreasing cortical tension ( Fig. 3f ), we use it at extremely low doses (see Methods section). Amazingly, it is sufficient to partially rescue spindle migration in 56% of the cases compared with 9% in non-injected mos−/− oocytes ( Fig. 4e,f , Supplementary Movies 4,5 ). We could not obtain a complete rescue, certainly due to the variability in the level of expression of the cRNAs injected. Indeed, the oocytes displaying a lack of spindle movement could either express too little cVCA (high tension, no spindle migration as in Fig. 1f blue curve) or too much cVCA (low tension, impaired spindle migration migration as in Fig. 1f red curve). Nevertheless, this rescue experiment further demonstrates that there is a direct link between spindle migration and cortical tension in this model. Altogether, we show that there is a range of tension, allowing spindle migration in mouse oocyte Meiosis I, and that this range is quite narrow ( Fig. 4g ). In our theoretical model, the force generator for spindle migration is myosin-II, pulling at spindle poles on the actin cage surrounding the microtubule spindle. The motor pulls when filaments emanating from the cortex and the actin cage overlap, creating a local stretching of the cortical actin thickening above the leading pole. This deformation is amplified when the spindle approaches the cortex ( Fig. 2a,b ), correlating to a high asymmetry in actin filament distribution ( Fig. 1a,c ), with more actin filaments overlapping between the leading pole and its above cortex, increasing the pulling force and the speed of spindle migration ( Fig. 2d ). In addition, at the end of Meiosis I when the spindle is in close proximity to the cortex, a Ran-GTP signal embarked by the chromosomes [30] induces local changes in cortical actin, leading to an Arp2/3-dependent cytoplasmic streaming that could also contribute to the acceleration of spindle movement [39] , [40] . When cortical tension is too high, the cortex cannot deform ( Supplementary Fig. 2a ) and the overlap does not increase ( Fig. 1b,c CK666-treated oocytes), thus the spindle stays centrally located ( Fig. 1d ). Similarly, when cortical tension is too low, myosin-II cannot properly pull on the cortex, as it is unable to sustain large pulling forces, preventing spindle migration ( Fig. 4a,b ). We can calculate from our model boundary values for cortical tension 0.01≤ k ≤0.1 nN μm −1 ( Fig. 4g ), the value measured in control oocytes being 0.034 nN μm −1 (ref. 9 ). Thus, cortical tension has to be fine-tuned within this range to promote spindle off-centering. It is interesting to wonder why such a narrow window of cortical tension has been conserved through evolution, as any variation around the appropriate value would give rise to a symmetric division or no division at all, possibly leading to oogenesis failure. A possibility is that cortical tension has an additional role after Meiosis I. For example, the cortex above the arrested Metaphase II spindle is more tense than the rest of the oocyte cortex [23] . It is possible that the decrease in cortical tension helps building an asymmetry between this region and the rest of the oocyte, preventing sperm entry where the oocyte is more tense and thus avoiding precocious DNA fusion between the sperm and the oocyte [41] . At meiosis resumption, oocytes start to break their link with follicular cells and become isolated cells [42] , implying that changes inside the oocyte can only come from within the cell as opposed to mitotic cells, which are able to read external constraints and respond to them [1] . Indeed, the precise regulation of cortical tension comes from the fact that the oocyte is able to trigger itself the decrease of cortical tension required for spindle migration by triggering the nucleation of an actin thickening that chases myosin-II from the cortex. This could be important to allow myosin-II to relocate at the poles of the actin cage and act as a force generator. To our knowledge, this is the first description of an F-actin network that is able to actively change the localization of myosin-II. The mechanism at play remains to be deciphered. One possibility could be that the nucleation of the cortical F-actin thickening creates an environment that is not favourable for myosin-II attachment to actin filaments, cortical filaments creating a very dense mesh [9] . In addition, photoactivation experiments point to the fact that the cortical actin network is far less dynamic than the cytoplasmic actin meshwork [9] . It is also possible that this cortical actin organization impedes on the localization of myosin-II: straight filaments nucleated by Formin-2 and Spire1/2 might have a better affinity for myosin-II than the Arp2/3-nucleated-branched filaments, in agreement with the fact that the activity of myosin-II is dependent on actin network architecture [43] . Alternatively, it is possible that the physical stress experienced by actin filaments modulates myosin-II recruitment. Indeed, in the amoeba Dictyostelium diskoideum , myosin-II is preferentially localized to actin filaments under tension [44] . Here, one could imagine that the filaments connecting the actin cage and the cortex, pulled by myosin-II, are under more stress than other cortical filaments and hence recruit more myosin-II, in an auto-amplificatory mechanism, increasing the depletion of myosin-II elsewhere in the cortex. One argument in favour of this hypothesis is that the so-called ‘actin cap’ above the Metaphase II spindle is more tense than the rest of the cortex [23] and is enriched in myosin-II [39] . Oocyte collection and microinjection and drug treatment Ovaries were collected from 11-week-old OF1 ( wt ) or mos−/− female mice. Competent oocytes were extracted by shredding the ovaries [45] and maintained in Prophase I arrest in M2+BSA medium supplemented with 1 μM milrinone [46] . At this stage, they were microinjected with cRNAs using an Eppendorf Femtojet microinjector. For rescue experiments in mos−/− oocytes, cRNAs encoding the cVCA were injected at a dilution of 50 ng μl −1 . Prophase I oocytes were kept for 2–3 h in Prophase I arrest to allow expression of fusion proteins. Meiosis resumption was triggered by releasing oocytes into milrinone-free M2+BSA medium. All live culture and imaging were carried out under oil at 37 °C. The stock solution of CK666 (gift from T Pollard and Calbiochem, ref. 182515) was diluted at 100 mM in dimethylsulphoxide and stored at −80 °C. It was used on oocytes at 200 μM starting from NEBD+3 h. Control experiments were performed in M2+BSA medium with equivalent dilutions of dimethylsulphoxide in separate dishes (the drug diffuses in the oil). Plasmids and in vitro transcription of cRNAs We used the following constructs: pspe3-GFP-UtrCH [18] , pRN3-histone-RFP [47] , pRN3-SF9-GFP [36] and pRN3-EB3-GFP [29] . We constructed pRN3-EzTD-mCherry-VCA by cloning the VCA domain of Wave2 amplified from pCS2-Wave2 (gift of A Gautreau) into pRN3-EzTD-mCherry (gift of S Louvet) [33] . We constructed also pRN3-histone-GFP by cloning histone-GFP from pcDNA3-histone-GFP (gift of G Halet) into pRN3. In vitro synthesis of capped cRNAs was performed using mMessage mMachine kit (Ambion) and RNeasy kit (Qiagen) following the manufacturer’s instructions [48] . cRNAs were centrifuged at 4 °C for 45 min at 20,000 g before microinjection. Live imaging Spinning disk images were acquired at 37 °C in M2+BSA medium using a Plan-APO x40/1.25NA objective on a Leica DMI6000B microscope enclosed in a thermostatic chamber (Life Imaging Service) equipped with a CoolSnap HQ2/CCD (charge-coupled device) camera (Princeton Instruments) coupled to a Sutter filter wheel (Roper Scientific) and a Yokogawa CSU-X1-M1spinning disk. Metamorph software (Universal Imaging) was used to collect data and ImageJ (NIH) to analyze and process data. Modelling of actin distribution in the oocyte We take the phenomenological assumption that actin filaments emanate from the actin cage tip and have an exponential distribution. The filaments grow in the cytoplasm and penetrate the cortex or grow in the cortex and are extracted in the cytoplasm. We call N(ℓ) the density of filaments at a given length ℓ . Then: , with ℓ 0 as the mean length of filaments in the cytoplasm, and with ℓ c as the mean length of the cortical part of the filaments. The density of filaments is thus given by: This density is plotted in Supplementary Fig. 1b . Assuming that the filaments emanating from the spindle poles grow slower when they penetrate inside the cortex than in the cytoplasm, in accordance with the fact that cortical actin and cytoplasmic actin define two different compartments in terms of dynamics [9] , we can postulate that the mean length of filaments in the cortex is shorter than in the cytoplasm, depending on the cortical tension. The length scale for the cytoplasmic actin filaments is a balance between polymerization and severing, so , with ℓ c as the mean length of filaments, penetrating the cortex, v p the polymerization speed (in m s −1 ) and α sev the severing rate (in s −1 ). Cortical tension should then decrease v p and the force-velocity relation for the polymerization against a load in the form: , with v p,0 as the growth rate for actin filaments in solution, k the cortical tension and k stall as the stall cortical tension at which the filaments cannot penetrate the cortex anymore. Thus, the length scale for the distribution of actin inside the cortex is given by that we can write to avoid negative values. The force is produced when the filaments emanating from the spindle poles overlap with the cortex, and the overlap is given by the mean length of overlap multiplied by the density of filaments. Measure of the GFP-UtrCH fluorescence intensity drop at NEBD Oocytes expressing GFP-UtrCH were imaged under the spinning disk every 30 min starting from Prophase I. The background was subtracted from the images using Metamorph software. Cytoplasmic and cortical integrated fluorescence intensities were measured and brought down to fluorescence intensity/pixels square. Then, the cytoplasmic fluorescence intensity/pixels square was divided by the cortical fluorescence intensity/pixels square at each time point to avoid discrepancies in the level of fluorescence due to differences in expression levels. The drop in GFP-UtrCH fluorescence intensity between NEBD-30 min and NEBD+30 min was calculated as the ratio between the two values at these time points. Actin distribution as a function of spindle position Control oocytes and oocytes treated with CK666 (refs 9 , 26 ) were imaged under the spinning disk every hour. A circular region of 8.4 μm 2 was used to measure the integrated fluorescence intensity above the lagging and leading poles 3, 2 and 1 h before polar body extrusion. For oocytes treated with CK666, the leading pole was defined as the closest pole from the cortex 3 h before polar body extrusion. The ratio between the fluorescence intensity above the leading pole and the fluorescence intensity above the lagging pole represents the asymmetry in actin distribution. The same region was used to measure the fluorescence intensity on the left and right side of the spindle (defined according to the leading pole), at the equatorial plane. The overall values were in the same range, oocytes treated with CK666 showing no difference in actin distribution in all directions and at all stages (one-way Anova, P -value=0.5722). Chromosome distance to the cell center was measured for each time point. In addition, for control oocytes, the fluorescence intensity of each region (leading, lagging, left and right) was normalized by the fluorescence intensity of the leading region for each time point ( Supplementary Fig. 1a ). Vesicle speed analysis Stream movies were acquired at a frequency of 500 ms for 5 min. Movies were then denoised using the Safir plugin for the Metamorph software (Universal Imaging), aligned and corrected for the bleaching using Fiji (NIH). Vesicles were then tracked using the Trackmate plugin for Fiji. The tracks were considered relevant when they exceeded 25 s. Cortical tension and viscosity measurements Measurements of cortical tension in Prophase I oocytes were performed using a viscous drop model and extrapolating the cortical tension by the pressure at which the cell enters the pipette [9] . Note that in the case of an interface with an elastic component, the tension is proportional to the elastic modulus (stiffness) of the system. For Prophase I wt and Ez overexpressing oocytes, the cortical tension was so high that the critical pressure could not be reached before blebs formed. Thus, to access a minimum value for critical pressure, we looked at which pressure we first saw bleb forming during cortex aspiration. The critical pressure would necessarily be bigger than this value, thus we used this pressure value as a ‘minimal’ critical pressure value. This allowed us to calculate a minimum value for cortical tension. For viscosity measurements, the zona pellucida of oocytes was removed using acid tyrod (pH=2.3). Oocytes were aspirated in a 50 μm diameter micropipette until they were completely inside the pipette ( Supplementary Fig. 1c ). Great care was taken that all oocytes stay inside the pipette for the same duration (around 100 s). They were then released and the shape recovery was recorded ( Supplementary Movie 6 ). The curve representing the evolution of the reduced diameter ( , with L the bigger diameter and l the smaller diameter, referred to as ‘relaxation ratio’) was plotted as a function of time and fitted as an exponential ( Supplementary Fig. 1d ). The characteristic time τ was extracted and the viscosity η was deduced from the formula: , with R c as the cell radius and k as the cortical tension. Statistical analysis Experiments were repeated at least three independent times and a sample of sufficient size was used. The statistical analysis was performed using GraphPad Prism version 6.00 for MacOS, GraphPad Software, La Jolla, California, USA, www.graphpad.com . Student’s t -tests (with Welch correction where indicated), χ 2 and one-way Anova or Kruskal–Wallis test were used with a confidence interval of 95%. In all figures, * corresponds to a P -value <0.05, ** to a P -value <0.005, *** to a P -value <0.0005 and **** to a P -value <0.0001. NS: not statistically Significant. How to cite this article : Chaigne, A. et al . A narrow window of cortical tension guides asymmetric spindle positioning in the mouse oocyte. Nat. Commun. 6:6027 doi: 10.1038/ncomms7027 (2015).